Clinically relevant copy number variations detected in cerebral palsy Cerebral palsy (CP) represents a group of non-progressive clinically heterogeneous disorders that are characterized by motor impairment and early age of onset, frequently accompanied by co-morbidities. The cause of CP has historically been attributed to environmental stressors resulting in brain damage. While genetic risk factors are also implicated, guidelines for diagnostic assessment of CP do not recommend for routine genetic testing. Given numerous reports of aetiologic copy number variations (CNVs) in other neurodevelopmental disorders, we used microarrays to genotype a population-based prospective cohort of children with CP and their parents. Here we identify de novo CNVs in 8/115 (7.0%) CP patients ( ∼ 1% rate in controls). In four children, large chromosomal abnormalities deemed likely pathogenic were found, and they were significantly more likely to have severe neuromotor impairments than those CP subjects without such alterations. Overall, the CNV data would have impacted our diagnosis or classification of CP in 11/115 (9.6%) families. Cerebral palsy (CP) is the most common cause of childhood physical disability, affecting ∼ 2.11 per 1,000 live births in high-resource settings [1] . CP arises from a non-progressive pathology that affects the developing brain either pre-, peri- or postnatally. Some of the established risk factors for CP include prematurity, intra-uterine growth restriction (IUGR), intra-uterine infections, birth defects and neonatal encephalopathy of various causes including perinatal asphyxia [2] , [3] , [4] . Recent studies suggest that birth asphyxia explains <10% of cases of neonatal encephalopathy [5] . Furthermore, there is tremendous variability in outcomes for any given risk factor, suggesting that some children may have an inherent higher susceptibility to CP. The consensus definition of CP [6] includes associated co-morbidities, such as epilepsy, communication impairment, sensory impairments or cognitive deficits, which greatly contribute to the associated health burden for children and families. CP can be classified by neurological subtype as well as by several functional classification systems. The neurological subtype stratification is based on the topographic distribution of affected limbs and the predominant quality of the observed motor impairment, grouping CP into subtypes: spastic quadriplegia, spastic diplegia, spastic hemiplegia, dyskinetic or dystonic, ataxic or hypotonic, or mixed. The motor severity can be described using the Gross Motor Function Classification System (GMFCS), which uses scores that range from most able (level I) to least able (level V) [7] . Twin and family studies suggest a genetic contribution to some CP [8] , [9] . Consanguineous families carrying recessive mutations in the glutamate decarboxylase 1 ( GAD1 ) gene have been described resulting in impaired production of γ-aminobutyric acid [10] . Treatment with drugs that potentiate γ-aminobutyric acid (for example, baclofen and benzodiazepine) ameliorate muscle rigidity and spasticity in these individuals, and have also been more generally used in CP [11] . Microdeletions of KANK1 have been identified in nine individuals with quadriplegia and intellectual impairment in a four-generation family [12] . Neuroimaging revealed brain atrophy and ventriculomegaly [13] , consistent with KANK1 ’s role in neuronal signalling and adhesion. Other studies have identified autosomal recessive variants in the adaptor protein complex 4 family ( AP4B1 , AP4E1 , AP4M1 and AP4S1 ) [14] , [15] of molecules involved in neuronal polarity [16] . Gene-based association studies testing for the potential role of common genetic variants in CP have not yet revealed bona fide risk loci [15] . To date, the literature on the genetic predisposition to CP has focused on selected patient populations with positive family history, dysmorphic features or atypical clinical features such as normal brain imaging. Routine genetic studies are not yet recommended in the diagnostic assessment of children with CP, especially in children where other risk factors are identified [17] . 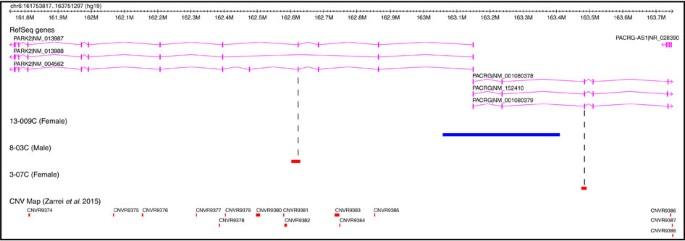Figure 1: CNVs affectingPARK2andPACRG. Thede novoduplication in patient 13-009C impacting bothPARK2andPACRGis illustrated by the blue bar above. Inherited deletions (denoted by the red bars) have been identified in exon 4 ofPARK2(NM_004562.2) in subject 8-03C and in exon 4 ofPACRG(NM_152410.2) in subject 3-07C. The recognition of the importance of de novo and rare inherited copy number variations (CNVs) in the clinical manifestations of a growing list of neurodevelopmental conditions ( Table 1 ) prompted us to test whether genomic abnormalities might similarly be observed in CP [18] . Our initial hypothesis was that de novo CNVs would be seen in an unselected cohort of children with CP more frequently than in the general population. Here we identify clinically relevant de novo and rare inherited CNVs at a comparatively high frequency that contributes to the aetiology of CP. Table 1 De novo CNV rates in related neurodevelopmental conditions. Full size table Clinically relevant variants Following our rigorous quality control procedure for CNV detection, 147 probands (81 males and 66 females) and 282 parents were used for the subsequent genomic analysis. The clinical characteristics of these children are described in Table 2 and specific cases are described in detail below. From this data, we identified 412 rare CNVs (in <0.1% of our population controls) in the probands ( Supplementary Data set 1 ). We compared the average number of unannotated calls and average CNV size between CP subjects and parents and found no significant difference for either of these measures using an unpaired Student’s t -test (two-tailed P values are 0.22 and 0.49, respectively) ( Supplementary Table 1 ). Among our samples were 115 complete parent–child trios (64 males and 51 female probands) that yielded sufficiently high-quality data allowing assessment of the segregation status of CNVs. Potentially contributory de novo or rare inherited CNVs were found in 11/115 families ( Table 3 ) and each of these was validated using the SYBR Green-based real-time quantitative PCR assay [19] . The clinical characteristics of these individuals are summarized in Supplementary Data set 2 . The potential clinical impact of CNVs was determined by comparison with the Database of Genomic Variants [20] and clinical CNV databases [21] . Table 2 Clinical characteristics of CP probands. Full size table Table 3 Summary of clinically relevant CNVs. Full size table For those four individuals (4-13C, 10-032C, 10-012C and 13-026C) with large (>5 Mb) CNVs deemed pathogenic or likely pathogenic and discussed in detail below, we tested whether they were more likely to have severe motor impairments. We examined the GMFCS scores provided at the time of registration for 103 of the probands and classified them as having mild-moderate (GMFCS I–III) or severe (GMFCS IV–V) motor impairments. One of the 78 cases with a GMFCS from I–III had a large de novo CNV (13-026C), while 3 of 25 with a score of IV or V had a large de novo variant. Using a two-tailed Fisher’s exact test, we confirmed that individuals with large CNVs were more likely to be severely impaired ( P =0.04). De novo CNVs De novo CNVs were identified in 8/115 (7.0%) trios and 4/115 (3.5%) of these subjects carried massive chromosomal structural abnormalities, which were likely the cause of CP, an associated disorder misdiagnosed as CP, and/or other co-morbidities in these individuals. Female 4-13C with dyskinetic CP—choreoathetotic subtype (GMFCS IV) carried a 74 Mb de novo duplication (371 genes; 2p25.3-2p13.1) and a 31 Mb de novo deletion (165 genes; Xp22.33-Xp21.2), suggestive of an unbalanced translocation. Her birth was induced at 39 weeks and she needed to be resuscitated. Magnetic resonance imaging identified a nonspecific bilateral white matter signal abnormality, bilateral cortical dysplasia in Sylvian areas and hypoplasia of the anterior falx cerebri. Female 10-032C with spastic quadriplegia (GMFCS V) carried de novo hemizygous deletions of 25.5 Mb (134 genes; 4p16.3-4p15.2) and 8.1 Mb ( KANK1 and 38 other genes; 9p24.3-9p24.1). Born at 34 weeks, she was 1.63 kg at birth with a head circumference of 27.5 cm and showed evidence of IUGR. Her mother had previous miscarriages and likely carries a balanced translocation. A cranial computed tomography scan identified improper formation of the subarachnoid space and hypoplasia. She is cognitively impaired, has seizures and severe scoliosis. Male 10-012C with spastic quadriplegia (GMFCS IV) has a 3.1 Mb de novo deletion (9 genes; 2p25.3), an adjacent de novo 12.1 Mb duplication (43 genes; 2p25.3-2p24.3), as well as a 43 kb de novo microdeletion affecting RAPGEF1 at 9q34.13. He was born at 40 weeks by spontaneous vaginal delivery, and exhibited motor and developmental problems and an ultrasound identified hydrocephalus. He was non-communicative, had visual impairment and strabismus. Male subject 13-026C, with dyskinetic CP—choreoathetotic subtype phenotype (GMFCS II)—was found to carry 5.8 Mb de novo deletion (18 genes) at 15q11.2-15q13.1 encompassing the type-I deletion associated with Angelman syndrome. The child was non-verbal, had cognitive impairments, and seizures before 25 months, but interestingly was not described as being ataxic. At age 5 years, his diagnosis was changed from CP to Angelman syndrome, as would be predicted by the microarray findings. A fifth subject, male 6-06C, with right spastic hemiplegia (GFMCS I) had a 2.8 Mb de novo duplication (20 genes; 22q13.31) characterized as being likely pathogenic. This CNV is below our 5 Mb cutoff described above and it affects an under-characterized region of the genome, so for now it is not yet deemed pathogenic. However, the large number of genes affected and its de novo occurrence place it in the category of having ‘likely clinical consequence’. His mother was hospitalized once during pregnancy for dehydration and gestational thrombocytopenia. The child was born at 39 weeks gestation with signs of neonatal encephalopathy. A computed tomography scan undertaken within 1 week of birth detected an ischaemic lesion in the frontoparietal area (both cortical and subcortical) around the left Sylvian artery. The three remaining CP cases carried smaller de novo CNVs, each characterized as a Variant of Unknown Significance due to a paucity of published reports regarding duplications of these genes [22] : female 13-009C with spastic quadriplegia (GMFCS V), female 4-10C with spastic diplegia (GMFCS I) and male 13-016C with dyskinetic CP (GMFCS V) had a 351 kb duplication (involving the first exon of PARK2 and the first two exons of PACRG ) ( Fig. 1 and below), a 48 kb duplication (affecting HSPA4 ) and 29 kb deletion (upstream of WNT4 ), respectively. Female 13-009C had signs suggestive of an acute intrapartum hypoxic event and needed resuscitation at birth. A head ultrasound identified diffuse oedema and slit-like ventricles consistent with hypoxic-ischaemic encephalopathy. Female 4-10C had no apparent prenatal or perinatal risk factors or other co-morbidities, but 13-016C experienced prenatal risk factors for CP and was born by emergency C-section at 24 weeks. A magnetic resonance imaging identified a stage II intraventricular haemorrhage (illustrating bleeding inside the ventricles) and diffuse white matter injury (as expected given prematurity). Without additional genetic findings in unrelated patients, such variants are of uncertain clinical relevance. Figure 1: CNVs affecting PARK2 and PACRG . The de novo duplication in patient 13-009C impacting both PARK2 and PACRG is illustrated by the blue bar above. Inherited deletions (denoted by the red bars) have been identified in exon 4 of PARK2 (NM_004562.2) in subject 8-03C and in exon 4 of PACRG (NM_152410.2) in subject 3-07C. Full size image Rare inherited CNVs Rare inherited CNVs affecting loci of known clinical genetic significance were detected in 3/115 (2.6%) of additional families. CP case 8-02C has spastic diplegia (GMFCS I) and carried a 2.1 Mb maternally inherited microdeletion (18 genes; 1q21.1-1q21.2), which exhibits variable phenotypic expression [23] , [24] . The prenatal and perinatal insults experienced likely caused CP, and the 1q21.1 microdeletion likely contributed to other complications such as IUGR and vision problems. Case 10-027C with spastic right hemiplegia (GMFCS I) carried a 1.4 Mb maternally inherited duplication (15 genes; 16p13.11), which may have contributed to her CP-associated co-morbidities of deficits in communication abilities [25] . Female 10-006C had spastic right hemiplegia (GMFCS II) and a paternally inherited duplication affecting part of the X-linked DMD muscular dystrophy gene, which is predicted to be likely benign. We also identified de novo and rare inherited CNVs affecting genes ( PARK2 , PACRG and HSPA4 ) involved in the unfolded protein response to endoplasmic reticulum stress, potentially providing insight into genetic and environmental interplay in CP ( Fig. 1 ). Three unrelated patients carried CNVs affecting the PARK2/PACRG locus, two overlapping genes co-regulated with a common bidirectional promoter [26] . In addition to the 351 kb duplication affecting the first exon of PARK2 and the first three exons of PACRG in case 13-009C described above, male 8-03C with spastic quadriplegia (GMFCS IV) and female 3-07C with spastic left hemiplegia (GMFCS II) carried a 26 kb deletion of exon 4 in PARK2 and a 14 kb deletion of exon 4 in PACRG , respectively. All three of these subjects experienced some form of pre-, peri- or postnatal insult, which likely led to their CP. Case 4-10C with spastic diplegia (GMFCS I) had a de novo 48 kb duplication affecting HSPA4 (mentioned previously), but no other risk factors for CP. Mutations in PARK2 are among the most common causes of autosomal recessive early-onset Parkinson’s disease and haploinsufficiency of the gene has also been shown to be a risk factor of familial forms [27] . PARK2 plays an important role in the ubiquitin–proteasome system in the endoplasmic reticulum, a process that targets proteins for destruction. PACRG, the Parkin co-regulated gene product, forms a complex with heat shock proteins (including HSPA4) and other chaperones to suppress cell death in response to an accumulation of unfolded protein. Given our CNV finding affecting these endoplasmic reticulum genes in CP, we speculate that a developmental insult(s) could perhaps elicit an unfolded protein response from prosurvival to the damaging pro-apoptotic phase elevating CP risk. It has been shown that immature neurons and preoligodendrocytes, which contribute to white matter formation, are particularly vulnerable to apoptosis as a result of endoplasmic reticulum stress [28] . Our genome-wide analysis yields new results indicating that large chromosomal abnormalities can be involved in CP. Prompted by our observations, we found deep in the literature an earlier study that used karyotyping to identify chromosomal anomalies in 8/100 (8%) individuals with CP [29] . The role of these anomalies in the pathogenicity of CP would require further assessment since in 6/8 cases the rearrangements were balanced or inherited, and one had 46, XYY aneuploidy, which is not known to be associated with CP. Most interestingly, the remaining subject had the Angelman syndrome deletion (15q11-q12) similar to 13-026C in our study. A recent microarray study of 52 CP families ascertained to be cryptogenic (no known aetiology) described 7/52 (13%) subjects as carrying de novo CNVs deemed pathogenic (one affecting a locus, KANK1 , found in our study and others) [30] . In our trio-based analysis, 10/101 individuals for which we had relevant data were cryptogenic, and 1/10 (10%) of these carried a de novo potentially clinically relevant CNV. A separate study of 50 unselected CP families failed to detect any de novo CNVs, but did find that ∼ 20% had a rare inherited CNV(s) of potential clinical relevance to the patient [31] . Recent exome sequencing studies of families [32] , [33] have also identified de novo sequence-level variants in CP subjects in some genes (for example, AGAP1 , L1CAM, PAK3, TENM1 and TUBA1A ) with potential functional relevance to the disorder. Two of these CP candidate genes ( AGAP1 and TENM1 ) [33] found by sequencing are also affected by CNV loci found in our study. As with our findings at the PARK2 locus ( Fig. 1 ), further replication experiments, however, are required to determine the pathogenicity of these genes before assigning clinical impact in CP. Taken together, there is a surge of new CNV data, and sequencing results that suggests a genomic basis for CP needs to be considered. In our systematic study, we determined a 7.0% de novo CNV rate in a population-based CP cohort, and ∼ 10% of the families studied carried clinically relevant CNVs that either explain the aetiologic basis of CP or possibly account for associated medical complications. The differences in our findings compared with other studies are likely due to the small samples sizes so far examined and different ascertainment strategies for CP, both being compounded by what appears to be a genetically heterogeneous disorder. Notwithstanding these complexities, for the majority of families in Table 3 , having the genetic data early would have enabled the recognition of a specific aetiology/diagnosis facilitating more accurate management, and counselling regarding recurrence risk. For example, case 13-026C was eventually clinically diagnosed with Angelman syndrome at age 5 years and had microarray analysis been performed earlier, his family would have received more accurate information about the natural history of his diagnosis (there is minimal, if any, speech development in Angelman syndrome). Similarly, in cases 4-13C, 10-032C and 10-012C carrying large CNVs aetiologic for the CP, a more accurate attribution of cause and genetic counselling would have ensued. In our experience, the remaining seven CP cases in Table 3 would also have been seen in clinical genetics and directed to the appropriate specialist. Importantly, finding another primary diagnosis (for example, microarray-based detection of chromosomal abnormalities and Wolf–Hirschhorn syndrome in 10-032C) does not negate a diagnosis of CP. A complete understanding of the effects of genotypes and environmental stressors on the clinical presentation(s) and manifestations of CP will require larger studies. In light of our new findings, however, we recommend that genomic analyses, in particular, high-resolution microarrays as a first tier and ultimately whole-genome sequencing, be integrated into the standard of practice for diagnosis and clinical categorization of CP. Participant selection We recruited 161 individuals with a CP diagnosis made by a paediatric neurologist, developmental paediatrician or physiatrist to form a population-based cohort from nine rehabilitation centres from the Canadian provinces of Alberta, Quebec and Ontario; 293 parents were also collected. Informed consent was obtained from parents and the study was approved by the Research Ethics Boards at Holland Bloorview Kids Rehabilitation Hospital, the University of Alberta and McGill University. Detailed standardized information regarding the child’s CP phenotypic profile including subtype, motor severity, medical co-morbidities, prenatal and perinatal factors were recorded. Microarray genotyping and quality control procedures DNA was extracted from saliva samples obtained from each proband and their biological parents. These samples were genotyped on the Illumina HumanOmni2.5-8 (San Diego, CA, USA) at The Centre for Applied Genomics in Toronto using established protocols [34] , [35] . Samples were required to have a minimum call rate of 0.95. The s.d. for the LRR (log R ratio) and BAF (B allele frequency) for an individual sample were required to be within the mean±three times the s.d. for the entire cohort for each of these criteria. Any sample outside this range was removed from further analysis. CNV calls were made using four different CNV detection algorithms: iPattern [36] , PennCNV [37] , QuantiSNP [38] and CNVPartition [36] . CNVs on autosomes required calling by at least two algorithms with one being either iPattern or PennCNV. CNV calls made on the X chromosome were only identified using iPattern and PennCNV and both algorithms were required to generate a stringent call. Very large CNVs were sometimes fragmented on account of both technical limitations of the array and the saliva samples used. As a result, all large CNVs were manually inspected and, if found to be fragmented, the calls were merged and sizes confirmed by examining the probe intensities and allele frequencies in the region ( Supplementary Fig. 1 ). Parent–child relationships were confirmed using PLINK [39] . All relevant microarray data have been deposited in the Gene Expression Omnibus and can be accessed using Gene Expression Omnibus accession number GSE70374 . Ancestry determination The ancestry of the 147 cases successfully genotyped on the HumanOmni2.5-8 were determined using HapMap3 samples (CEU, TSI, YRI, JPT, CHD and CHB) genotyped on Genome-Wide Human SNP Array 6.0 as the reference set ( Supplementary Data set 3 ). Single-nucleotide polymorphism (SNP) genotypes for both the HapMap and case samples were extracted and formatted for analysis using PLINK v1.90b2. After excluding the SNPs on the sex chromosomes, ambiguous SNPs, and those overlapping the major histocompatibility complex region, SNPs were filtered based on their minimum allele frequency (MAF) using the PLINK toolkit [39] . For each of the sets, all SNPs that had a genotyping rate <95% or where the MAF <5% were excluded. The SNPs common to the two platforms were extracted and the two data sets were combined. This time, all SNPs with a genotyping rate <95% or where the MAF <5% in the combined data set were removed. Linkage disequilibrium-based pruning of the autosomal SNPs with parameters 50 (window size), 5 (step) and 0.25 ( r 2 threshold) yielded 96,023 SNPs for the analysis. Population stratification and outlier detection were performed by multidimensional scaling analysis as implemented in PLINK. The top two principal components were then plotted using a custom R script ( Supplementary Fig. 2 ). Rare variant detection Rare variants were identified as those present in <0.1% of our population controls using <50% reciprocal overlap [40] . They were required to overlap (>75%) copy number stable regions of the genome [41] , be called by at least five successive probes, and exceed 10 kb in size. Our primary control data sets included 2,988 population control samples obtained from the KORA (Cooperative Research in the Region of Augsburg) [42] and the COGEND (Collaborative Genetic Study of Nicotine Dependence) [43] , which were genotyped using the Illumina Human OMNI 2.5M-Quad microarray. We subsequently compared our CNV calls with those obtained from other population control individuals to further refine our list of rare variants. We utilized additional population control samples including 1,234 from the Ontario Heart Research Institute [44] and 1,123 from the POPGEN [45] (both cohorts were run on the Affymetrix 6.0 microarray); 1,769 controls from the SAGE consortium [46] , 433 controls from the Ontario Family Colorectal Cancer Registry [47] and 2,566 from the Health, Aging and Body Composition study [48] (from the Illumina 1M microarray); and 873 from the Ontario Population Genetics Platform [49] (from the CytoScan HD). Validation of CNV findings CNVs of potential clinical relevance ( Table 3 ; Supplementary Table 2 ) were confirmed in patient and parental samples (where available) using a SYBR Green-based real-time quantitative PCR assay. Primer3 software v. 0.4.0 ( http://bioinfo.ut.ee/primer3-0.4.0/ ) was used to generate primer sequences that produce a PCR product of 90–140 bp. We also designed control primers to amplify a region of the FOXP2 locus. NA10851 and NA15510 were used as our male and female controls and each experiment was performed in triplicate. Primer sequences used to amplify candidate regions can be found in Supplementary Table 3 . Control sample permissions We obtained the KORA, COGEND and Health ABC (HABC) control cohorts along with permission for use, from the database of Genotypes and Phenotypes found at http://www-ncbi-nlm-nih-gov.myaccess.library.utoronto.ca/gap through accession numbers phs000169.v1.p1 (Whole Genome Association Study of Visceral Adiposity in the HABC Study), phs000303.v1.p1 (Genetic Epidemiology of Refractive Error in the KORA Study) and phs000404.v1.p1 (COGEND; The Genetic Architecture of Smoking and Smoking Cessation). The Division of Aging Biology and the Division of Geriatrics and Clinical Gerontology, National Institute on Aging provided support for the ‘Center for Inherited Disease Research Visceral Adiposity Study’. HABC Study Investigators provided study coordination and assistance with phenotype harmonization and genotype cleaning. The National Eye Institute provided support for the KORA data set that was obtained from the NEI Refractive Error Collaboration Database. Genotyping of the COGEND samples was conducted at the Center for Inherited Disease Research and support was provided by 1 X01 HG005274-01. The Gene Environment Association Studies (GENEVA) Coordinating Center (U01HG004446) provided study coordination and assistance with genotype cleaning for these samples. The COGEND (P01 CA089392) and the University of Wisconsin Transdisciplinary Tobacco Use Research Center (P50 DA019706 and P50 CA084724) provided the support for sample collection for the COGEND samples and data sets. The contents of this article are solely the responsibility of the authors and do not necessarily represent the official views of the NIH. Accession codes: All relevant microarray data has been deposited in the Gene Expression Omnibus (GEO) and can be accessed using GEO accession number GSE70374 . How to cite this article: Oskoui, M. et al . Clinically relevant copy number variations detected in cerebral palsy. Nat. Commun. 6:7949 doi: 10.1038/ncomms8949 (2015).